Structured cone arrays for continuous and effective collection of micron-sized oil droplets from water Environmental protection agencies and the petroleum industry require effective methods to separate micron-sized oil droplets from water. However, for most existing separation methods, phase separation occurs in the oil–water mixture. The remaining micron-scale oil droplets, which are not affected by phase separation, are difficult to handle with conventional methods on a large scale because of either a lack of separation ability or drawbacks in throughput capacity. Here we develop an oleophilic array of conical needle structures for the collection of micron-sized oil droplets, inspired by the collection of similar sized water droplets on conical cactus spines. Underwater, these structures mimic cacti and can capture micron-sized oil droplets and continuously transport them towards the base of the conical needles. Materials with this structure show obvious advantages in micron-sized oil collection with high continuity and high throughput. Environmental protection and economic development have increased the demand for materials that can effectively separate oil–water mixtures [1] , [2] , [3] . The petroleum industry also requires novel oil–water separation methods to improve oil recovery [4] , [5] . In the field of oil–water separation, materials with special wettabilities and micro- and nanostructures have attracted the attention of many researchers; these materials include polymer-coated meshes [6] , [7] , [8] , hydrogel-coated meshes [9] , polymer networks [10] and surface-modified meshes [11] , [12] , [13] , [14] , although for these methods, phase separation occurs readily in the oil–water mixture. If the mixture is undisturbed for a period of time, it will separate by itself to form a water layer and an oil layer. However, oil–water mixtures from practical applications contain many micron-sized oil droplets, which are not affected by phase separation and cannot be separated through these methods. To date, although there are a few methods capable of separating micron-sized oil droplets [15] , [16] , [17] , high continuity or high throughput remains difficult to achieve. The collection of micron-sized water droplets by cacti relies on the directional transport of liquid droplets [18] , which is also applied in many applications, including fog harvesting [19] , [20] , filtration [21] , condensers [22] and microfluidic devices [23] , [24] , [25] . The micron-sized water droplets can be driven by the conical structure during water deposition [18] . Micron-sized oil droplets in water and micron-sized water droplets in air are similar, so we can move the cactus-inspired system underwater. Thus, here we fabricate a novel oleophilic conical needle structure that can successfully separate micron-sized oil droplets from the oil–water mixture and can drive the droplets towards their base; in this way, continuous and effective collection of micron-sized oil droplets from water is achieved. Collection of micro oil droplets on single Cu-based needles To test the capability of a single conical needle to collect micron-sized oil droplets, we fabricated a series of conical Cu-based needles from commercial Cu wire with a diameter of 0.5 mm (see details in the Methods section and in Supplementary Fig. S1 ). The oil–water mixture was sprayed onto the conical needles, which were already immersed in water ( Supplementary Fig. S2 ). The oil–water mixture contained oil droplets smaller than 10 μm ( Supplementary Fig. S3 ); these droplets are difficult to separate using other existing methods with high throughput. Several key frames from videos taken throughout the collection process are shown in Fig. 1a,b . On the smooth Cu-based needle, the collected oil droplets grew through frequent coalescence and slowly moved towards the base of the needle. However, on the rough Cu-based needle, the collected oil droplets could be driven very quickly towards the base of the needle. The difference between these two phenomena is caused by the different roughnesses. 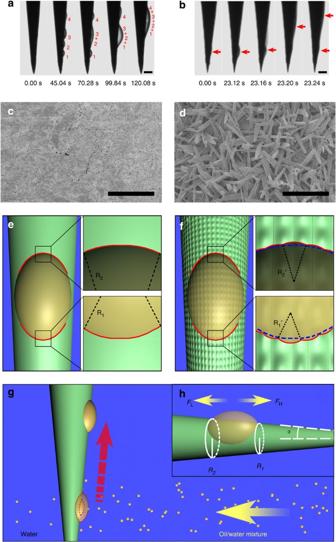Figure 1:In situobservation and schematic of the oil collection process. (a)In situobservation of the oil collection process on a smooth Cu-based needle. The collected oil droplets moved upwards as they combined. (b)In situobservation of the oil collection process on a rough Cu-based needle. The collected oil formed a growing droplet (nanolitre to picolitre scale), and when the droplet was driven upwards, a fresh surface was left for another cycle. (c) SEM image of a smooth Cu-based needle. (d) SEM image of a rough Cu-based needle. (e,f) Top views of TCLs and mechanism of roughness enhancement. The smooth needle is on the left side, the rough needle is on the right side and the red lines indicate the TCLs. (g) Schematic of the oil collection process. Micron-sized oil droplets deposit on the needle. The collected oil droplet grows and is then driven upwards. (h) Estimation of forces when a droplet is in the clam-shell shape.FLis the vertical component of the force induced by the Laplace pressure.FHis the hysteresis resistance force. Scale bars, (a,b): 30 μm; (c,d): 5 μm. Figure 1: In situ observation and schematic of the oil collection process. ( a ) In situ observation of the oil collection process on a smooth Cu-based needle. The collected oil droplets moved upwards as they combined. ( b ) In situ observation of the oil collection process on a rough Cu-based needle. The collected oil formed a growing droplet (nanolitre to picolitre scale), and when the droplet was driven upwards, a fresh surface was left for another cycle. ( c ) SEM image of a smooth Cu-based needle. ( d ) SEM image of a rough Cu-based needle. ( e , f ) Top views of TCLs and mechanism of roughness enhancement. The smooth needle is on the left side, the rough needle is on the right side and the red lines indicate the TCLs. ( g ) Schematic of the oil collection process. Micron-sized oil droplets deposit on the needle. The collected oil droplet grows and is then driven upwards. ( h ) Estimation of forces when a droplet is in the clam-shell shape. F L is the vertical component of the force induced by the Laplace pressure. F H is the hysteresis resistance force. Scale bars, ( a , b ): 30 μm; ( c , d ): 5 μm. Full size image To quantify the capability of a single needle for oil collection, we found a method to measure this capability. The needles were suspended from a micro-electromechanical balance system while they were immersed in water. Before the spraying of the oil–water mixture, the balance system measures the combined forces of gravity and buoyancy. After the spraying of the oil–water mixture, the oil droplets collected under water experience larger forces from buoyancy than from gravity, so the resultant force measured by the balance system will be reduced and the reduction will reflect the amount of collected oil. The weight changes were measured after spraying for 30 s. The weight changes on smooth Cu-based needles were −1.92±0.30 mg, and those on rough Cu-based needles were −4.98±0.26 mg. It was obvious that the rough needles collected oil more efficiently. Three steps were found during oil collection on the surface of the rough conical needle: deposition, growth and self-driven motion ( Fig. 1b,g ). The driving force and the resistance force were the primary forces in the oil collection process. The droplets on the conical structure were subjected to the directional force induced by the difference in the Laplace pressure (curvature gradient) [20] , [26] . In most cases, for droplets on a solid surface, contact angle hysteresis resulting from capillary forces would exist [19] , [20] , [27] and oppose the motion of the droplets. Particularly for droplets on the sub-millimetre scale, the hysteresis effect is so predominant that it is usually difficult to move the droplet [20] , [28] . In this case, for motion, a larger driving force is needed to overcome the significant hysteresis force; this force can be achieved by integrating multiple gradients or by increasing the singular gradient effect with roughness. Figure 1h shows that the forces on the oil droplet were the vertical component of the force induced by the difference in the Laplace pressure ( F L ) and the hysteresis resistance force ( F H ). The micron-sized oil droplets in the oil–water mixture deposited on the surface when they came in contact with the conical needles. Thereafter, the oil droplets grew through frequent coalescence. When the F L acting on the droplets was large enough, the droplets moved upwards quickly ( ∼ 2 mm s −1 ) and left a clean surface, which could start another collection cycle. As a result, the conical needle could continuously collect oil from the oil–water mixture, as shown in Supplementary Movie 1 . In addition, Supplementary Movie 2 shows simulations of these steps: deposition, growth and self-driven motion. Collection of micro oil droplets on single PDMS needles As it was complicated to make an array of the conical Cu needles, we chose to fabricate conical needles from polydimethylsiloxane (PDMS). PDMS is intrinsically oleophilic and is easy to mould. 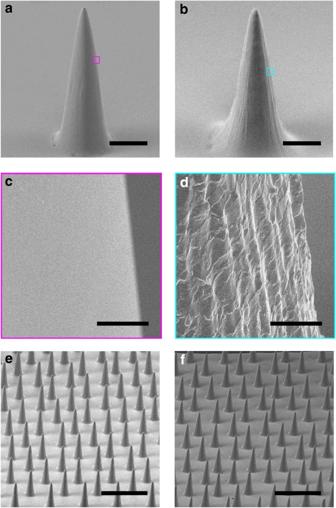Figure 2: SEM images of conical PDMS needles and arrays. (a) SEM image of a smooth PDMS needle. (b) SEM image of a rough PDMS needle. (c) Enlarged image of a smooth PDMS needle. (d) Enlarged image of a rough PDMS needle. After spraying the oil–water mixture for 30 s, the needle in (b) showed a larger weight change (−3.66±0.42 mg) than the needle in (a) (−2.61±0.53 mg). (e) SEM image of an array of smooth PDMS needles. (f) SEM image of an array of rough PDMS needles. Scale bars, (a,b): 100 μm; (c,d): 5 μm; (e,f): 500 μm. Figure 2a,b shows the scanning electron microscope (SEM) images of single PDMS needles. The surfaces of these PDMS needles are covered with spaced ridges ( Fig. 2d ). The widths of the ridges fit a random distribution of around one micron. Smooth and rough single PDMS needles can also be made into arrays ( Fig. 2e,f ), as shown below in more detail. The weight changes after spraying for 30 s on smooth PDMS were −2.61±0.53 mg, and the changes on rough PDMS were −3.66±0.42 mg. It was obvious that the rough needles could collect oil more efficiently. This result was consistent with the previous experiments on Cu-based needles. Figure 2: SEM images of conical PDMS needles and arrays. ( a ) SEM image of a smooth PDMS needle. ( b ) SEM image of a rough PDMS needle. ( c ) Enlarged image of a smooth PDMS needle. ( d ) Enlarged image of a rough PDMS needle. After spraying the oil–water mixture for 30 s, the needle in ( b ) showed a larger weight change (−3.66±0.42 mg) than the needle in ( a ) (−2.61±0.53 mg). ( e ) SEM image of an array of smooth PDMS needles. ( f ) SEM image of an array of rough PDMS needles. Scale bars, ( a , b ): 100 μm; ( c , d ): 5 μm; ( e , f ): 500 μm. Full size image To summarize, the investigations above considered two variables of the collection surface: material and roughness. From the experiments with Cu-based and PDMS needles, it was conjectured that the ability to collect micron-sized oil droplets was not only present in special materials but was widely manifested in ordinary oleophilic materials. Importantly, there was no need to clean the surface of the conical needles for reuse. After one oil droplet was driven upwards, another droplet arose and grew in the same manner. This driving of the micron-sized oil droplets is very useful in oil collection. Once the oil droplets were driven upwards to the base of the conical needle, they formed a large droplet, which was easy to pump out macroscopically ( Supplementary Movie 3 ). Further applications of PDMS needle arrays Arrays of conical PDMS needles were applied for further massive oil collection. The ‘throughput’ and ‘efficiency’ are defined here to quantify the collection ability of the needle arrays. The volume of the oil–water mixture that can be treated per second per square centimetre is defined to be the ‘throughput’. The percentage of oil that can be collected from the oil–water mixture is defined to be the ‘efficiency’. A commercial sewing needle and an xyz-controlled system combined with a method for PDMS replication were used to fabricate the array. First, needle arrays with square and hexagonal grids of both smooth and rough needles were designed (see SEM images in Supplementary Fig. S4 ). The roughness of the structure was the same as that for the single PDMS needles described previously. The PDMS replica (with a size of 0.8 cm × 0.8 cm) was immersed under water at an angle before being sprayed with the oil–water mixture ( Fig. 3a ). Similar to the experiments on single conical needles (the oil droplets collected by a single conical needle are driven towards the base and form a larger macroscopic droplet), the collected oil droplets formed a large droplet and converged at the upper edge of the PDMS replica because of the buoyancy force under water ( Supplementary Movie 4 ). 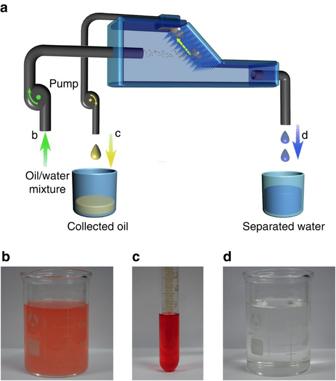Figure 3: Oil collection on PDMS needle arrays. (a) Schematic of the collection device. When the oil–water mixture flowed through the needle array, the oil in the mixture was collected by the conical needles, and the pure water flowed towards the other end of the device. (b) Oil–water mixture. (c) Collected oil. (d) Separated water, nearly no visible red oil was present. To facilitate observation, Oil Red O is added to the oil. Figure 3: Oil collection on PDMS needle arrays. ( a ) Schematic of the collection device. When the oil–water mixture flowed through the needle array, the oil in the mixture was collected by the conical needles, and the pure water flowed towards the other end of the device. ( b ) Oil–water mixture. ( c ) Collected oil. ( d ) Separated water, nearly no visible red oil was present. To facilitate observation, Oil Red O is added to the oil. Full size image To quantify the efficiency of the collection, the oil content in the oil–water mixture was measured before separation ( Fig. 3b ), and the result was defined to be V 0 . The oil content after the oil–water separation ( Fig. 3d ) was also measured and was defined to be V C . The difference between V 0 and V C can be considered as the volume of oil collected. The collection efficiency could be calculated from the formula: R(%)=(1−( V C / V 0 )) × 100%. The collection efficiencies for the four types of arrays were measured separately; the smooth square arrays had an efficiency of ∼ 93.7±2.3%, the smooth hexagonal arrays had an efficiency of ∼ 96.2±1.9%, the rough square arrays had an efficiency of ∼ 95.6±0.8% and the rough hexagonal arrays had an efficiency of ∼ 98.9±0.4% ( Supplementary Fig. S4 ). It was clear that the arrays with hexagonal grids have higher efficiencies than the arrays with square grids because the needle densities are larger. Rough needle arrays are more efficient because of the roughness enhancement, which is discussed below. Thus, we chose the rough hexagonal array for the following experiments and studied the effects of the separation between needles and the height of the needle arrays. A series of rough hexagonal arrays were fabricated with different needle separations and array heights (see SEM images in Supplementary Fig. S5 ). The needle separation in the arrays was from 500 to 250 μm ( Fig. 4a ), and the heights of the conical needles in the array were from 0 to 500 μm ( Fig. 4b ). It was obvious that both the needle separation and array height could affect the collection efficiency. Smaller needle separations and greater array heights can provide larger array densities and greater contact areas, and these properties are important for oil collection. 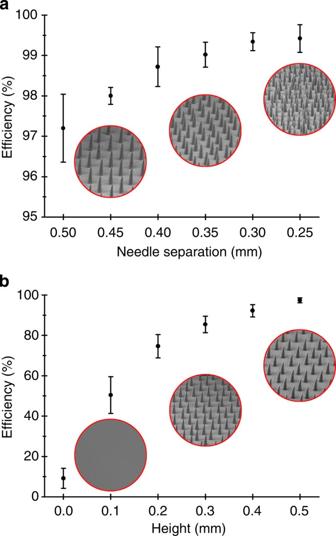Figure 4: Efficiencies of oil collection on PDMS needle arrays. (a) Efficiencies of needle arrays with different needle separations. The three inset SEM images are the arrays with needle separations of 0.50, 0.35, and 0.25 mm. A larger needle density provided a higher efficiency. (b) Efficiencies of needle arrays with different heights. The three inset SEM images are the arrays with heights of 0.0, 0.3, and 0.5 mm. Higher needles provided a larger efficiency. Each point represents the average efficiency of seven samples; the error bars indicate the standard deviation. Figure 4: Efficiencies of oil collection on PDMS needle arrays. ( a ) Efficiencies of needle arrays with different needle separations. The three inset SEM images are the arrays with needle separations of 0.50, 0.35, and 0.25 mm. A larger needle density provided a higher efficiency. ( b ) Efficiencies of needle arrays with different heights. The three inset SEM images are the arrays with heights of 0.0, 0.3, and 0.5 mm. Higher needles provided a larger efficiency. Each point represents the average efficiency of seven samples; the error bars indicate the standard deviation. Full size image To quantify the throughput for oil collection in the needle array, the parameters of the spray were changed. Needle arrays that were 0.8 cm × 0.8 cm in size were used. The major parameters that could be changed included the size of the syringe needles (different internal diameters), the flow velocity and the number of needles spraying simultaneously ( Supplementary Fig. S6 ). The effective usage area of the PDMS array was maintained at ∼ 0.125 cm 2 . The flow rate was changed from 0.009 ml s −1 to 0.141 ml s −1 . Accordingly, the throughput could be as much as 1.128 ml cm −2 s −1 . As the parameters changed, the efficiency was relatively invariable and high. Therefore, the throughput can be improved by changing the parameters. The improved throughput could provide potential industrial applications for large area arrays or with pipes instead of syringe needles. According to the sections on the collection of micron-sized oil droplets on single Cu-based needles and single PDMS needles, the ability to collect micron-sized oil droplets existed for both types of needles. The similarity in the results for single Cu-based and PDMS needles is reasonable. The ability to deposit oil is based on the intrinsic oleophilicity of these materials under water, and the conical structure induces the directional motion of the collected oil droplets. Therefore, the key qualities for continuous oil collection are oleophilicity and a conical structure. To validate this result, other oleophilic materials were tested in conical structures, including Au-coated needles, polyaniline-coated needles and rubbed polystyrene needles (see Supplementary Fig. S7 ). These needles can also continuously collect oil from an oil–water mixture. Based on the further applications of PDMS needle arrays, the collection efficiency of the PDMS needle array could be ∼ 99%. Almost no visible oil (which had been dyed red with Oil Red O) existed in the separated water ( Fig. 3d ). It was conjectured that many types of micron-sized oil droplets could be collected by this needle array. Accordingly, a variety of oil–water mixtures and organic solvent/water mixtures, including low-viscosity silicone, gasoline, vegetable oil, hexane and petroleum ether, were successfully separated through the same process. Thus, materials with conical structures may find potential applications in environmental protection, chemical engineering and the petroleum industry. The micron-sized oil droplets on single needles moved slowly on the smooth Cu needles towards the base through coalescence. However, on the rough Cu-based needles, the collected oil droplets could be driven towards the base very quickly. The difference between these two phenomena arises from the increased oleophilicity caused by the surface roughness when the droplets are in the Wenzel state [29] , [30] ; thus, the Laplace pressure is different on the conical structured needle ( Fig. 1e,f ). The convex structure of the rough needles modifies the oil–water–solid three-phase contact line (TCL) of the oil droplet. On the smooth needle, the Laplace pressures at the two opposite sides of the droplet can be represented as follows [19] , [20] : where R 1 and R 2 are the local radii of the TCLs at the two opposite sides, γ water is the surface tension of water and γ oil is the surface tension of oil. The Laplace pressure at the two opposite sides of the droplet can be written thus: where R ′ 1 and R 2 ′ are the local radii of the TCLs at the two opposite sides. On the rough needle, the TCLs are divided into several parts by the rough structures, and this division gives rise to the decreased local radius of the TCLs and the enlarged local curvatures. Therefore, the difference in the Laplace pressures (Δ P ′) is enlarged by the roughness: The enlarged difference in the Laplace pressures provides a larger driving force on the rough surface, or equivalently, the rough needle leads to smaller initial radii for the driven droplets. Thus, the rough needle can provide a larger fresh surface for oil collection. Because the fresh rough surface can collect oil droplets more efficiently than the smooth surface, the rough needle can collect oil faster. As is known, in air, water droplets can be driven by shape gradients [18] , [19] , [26] . In our research, this effect also exists for oil droplets under water. Figure 1h shows that the forces on the oil droplet were the vertical component of the Laplace Force ( F L ) and the hysteresis resistance force ( F H ). F L and F H can be represented as follows: where α is the semi-apex angle of the conical needle, V is the volume of the oil droplet, R 0 is the radius of the oil droplet, θ r and θ a are the receding and advancing contact angles, and R 1 and R 2 are the local radii at the two opposite sides of the droplet (see details in Supplementary Note ). The maximum of F H is constant when R 0 is invariable, and when the oil droplet grows, V and F L increase. Thus, if the oil droplet is not large enough, F L is smaller than the maximum of F H , and the droplet cannot move; as the droplet grows, once F L becomes larger than the maximum of F H , the oil droplet is driven towards the base of the needle. For the droplet 1+2+3+4 in Fig. 1a , the maximum of F H is ∼ 1.5 × 10 −6 N for R 1 ∼ 20 μm, R 2 ∼ 30 μm and V ∼ 60 pL; F L is ∼ 1.1 × 10 −6 N, and hence the oil droplet does not move by itself. For the droplet in Fig. 1b , the maximum of F H is ∼ 7.7 × 10 −7 N for R 1 ∼ 10 μm, R 2 ∼ 20 μm and V ∼ 6 pL; F L is ∼ 6.9 × 10 −7 N, but the roughness enhanced F L by decreasing R 1 and R 2 and making F L larger than the maximum of F H ; thus, the oil droplet could be driven upwards. In addition, the gravity and buoyancy forces can be neglected in principle because F L and F H are 10 −7 –10 −6 N and because the gravity force and buoyancy force are 10 −12 –10 −11 N. Rough needles can collect oil droplets more efficiently than smooth needles, and we found a method to quantify the roughness enhancement. A series of Cu-based needles with different roughnesses were fabricated ( Supplementary Fig. S8 ). The needle surfaces were covered with nanorods with different lengths and diameters. The lengths of the nanorods ranged from 0 to 6.7±0.5 μm, and the diameters were from 0 to 472±141 nm. The weight changes after spraying for 30 s were also measured and were from −1.92±0.30 to −4.95±0.22 mg ( Supplementary Fig. S9 ). These results were homologous with the roughness of the needles. The conical-apex angle also affects the collection efficiency. After spraying for 30 s, the weight changes on single conical needles with different conical-apex angles were measured; the changes were −4.40±0.18 mg at 10° and −5.43±0.22 mg at 15° and changed linearly ( Supplementary Fig. S10 ). The needles with larger conical-apex angles can collect oil faster. The faster collection occurs because of the larger conical-apex angle: if the conical-apex angle is larger, the F L in equation (4) equals F H at smaller volumes. Equivalently, larger conical-apex angles lead to smaller initial radii for the driven droplets. Thus, the needles with larger conical-apex angles can provide more fresh surfaces for oil collection. Therefore, the needles with larger conical-apex angles can collect oil droplets faster. In conclusion, a novel oleophilic conical needle material was successfully fabricated and demonstrated exciting oil collection properties in oil–water–solid three-phase systems. The conical needle can collect micron-sized oil droplets from the oil–water mixture and can achieve directionally controlled transport of micron-sized oil droplets. A conical needle array can continuously collect oil from an oil–water mixture with high efficiency and high throughput. Furthermore, other oleophilic materials with conical structures are expected to be usable for continuous oil collection. The introduction of stimuli-responsive polymers will also aid in the design of smart materials and in oil–water separation from oil-in-water emulsions. Fabrication of single conical needles In the process of fabricating single Cu-based needles, a simple electroetching process was used. Commercial Cu wire with a diameter of 0.5 mm was used as the raw material. Initially, burnished copper wires were immersed in an aqueous solution of 0.1 M CuSO 4 at room temperature. Then, the wires were electroetched at a voltage of 10 V, and the Cu wires were raised and lowered at a velocity of 0.1 mm s −1 for hundreds of cycles to form conical needles. The relatively smooth Cu-based needles were fabricated by immersing these as-prepared conical Cu needles in an ethanol solution of 1-hexadecanethiol (10 mM) for 15 min, then washing the wires with ethanol and drying the wires in air. The relatively rough Cu-based needles were fabricated by roughening the as-prepared conical Cu needles by immersing the wires in an aqueous solution of 1.0 M NaOH and 0.05 M Na 2 S 2 O 8 at room temperature for 15 min [11] , [14] , [31] . The reaction time for this stage could be changed to fabricate needles with different roughnesses. After being washed with water and then dried in air, the needles were further immersed in a solution of 1-hexadecanethiol in ethanol (10 mM) for 15 min; then, the needles were washed with ethanol and were dried in air ( Supplementary Fig. S1 ). In the process of fabricating single PDMS needles, commercial sewing needles were used to prick the surfaces of slices of polyethylene (PE) (with thicknesses of 1 mm), and PE slices with conical holes were obtained. Then, using a mature and widely applied technology [32] , [33] , PDMS was applied to replicate the conical holes, and PDMS replicas of smooth conical needles were formed. Moreover, if we rubbed the commercial sewing needles with sandpaper, the surfaces of the final PDMS replica needles exhibited a rough morphology. Experiments on single conical needles The conical needles were immersed in deionized water. Numerous micron-sized oil droplets were generated by stirring and ultrasonically treating the mixture of low-viscosity silicone (PMX200-5CS, Dow Corning) and deionized water (5:95, silicone:water, by weight). Supplementary Fig. S3 shows a microscope image of the micron-sized oil droplets with diameters ranging from 1 to 4 μm. The mixture was sprayed through the syringe needles onto our conical needles ( Supplementary Fig. S2 ). The entire process was recorded by the optical microscopy components of the OCA40 system. The weight changes were measured under the same conditions with the exception that the conical needles were suspended from the micro-electromechanical balance system of the DCAT 11. Fabrication and experiments on conical needle arrays The fabrication process for the needle arrays is shown in Supplementary Fig. S11 . Commercial sewing needles with conical-apex angles similar to that of the single conical needles were attached to a jet dispensing system. PE slices were pricked to form the hole array. PDMS (Sylgard 184, Dow Corning) was applied to replicate the surface of the hole array. The PDMS replicas exhibit the morphology of an array of conical needles. The oil–water mixture was sprayed onto the conical needle arrays ( Fig. 3a ); to facilitate observation, a small quantity of Oil Red O was added to the mixture. Instruments and characterization SEM images of the samples were obtained with a field-emission scanning electron microscope (JSM-6700 F, Japan). Experiments on single conical needles were performed on an OCA40 machine (Data-Physics, Germany). Micrographs were obtained with a Leica DM4000M microscope (Germany). The weight changes during the collection of oil on single conical needles were measured with a high-sensitivity micro-electromechanical balance system (Data-Physics DCAT 11, Germany). The conical hole arrays were fabricated with a jet dispensing system (Nordson EFD-PicoDot, USA). How to cite this article: Li, K. et al. Structured cone arrays for continuous and effective collection of micron-sized oil droplets from water. Nat. Commun. 4:2276 doi: 10.1038/ncomms3276 (2013).